The Gibberellin perception system evolved to regulate a pre-existing GAMYB-mediated system during land plant evolution Gibberellin (GA) controls pollen development in flowering plants via the GAMYB transcription factor. Here we show that GAMYB is conserved in Selaginella moellendorffii (lycophyte) and Physcomitrella patens (moss), although the former contains the GA signalling pathway, the latter does not. In the lycophyte, GA treatment promotes the outer wall development on microspores, whereas treatment with GA biosynthesis inhibitors disturbs its development. Contrary, in the moss, GAMYB homologue knockouts also produce abnormal spores that resemble Selaginella microspores treated with GA biosynthesis inhibitors and pollen grains of rice gamyb mutant. Moreover, the knockouts fail to develop male organs, instead ectopically forming female organs. Thus, before the establishment of the GA signalling pathway, basal land plants, including mosses, contained a GAMYB-based system for spore and sexual organ development. Subsequently, during the evolution from mosses to basal vascular plants including lycophytes, GA signalling might have merged to regulate this pre-existing GAMYB-based system. In flowering plants, gibberellin (GA) regulates the formation of the outer wall on pollen and is therefore essential for pollen development [1] , [2] , [3] . The outermost pollen wall, which is known as the exine or exospore, consists largely of sporopollenin, an organic polymer that is extremely resistant to degradation and is so durable that it has been found in microfossils that are over 500 million years old [4] , [5] , [6] . In rice, CYP703A3 is an essential enzyme in sporopollenin biosynthesis, and its expression is positively regulated by a transcription factor, GAMYB, which is controlled by the GA signalling pathway [1] , [7] , [8] . Previous anatomical and in silico studies suggest that, similar to flowering plants, present-day bryophytes, including mosses, and lycophytes (lycopods) contain sporopollenin-containing outer walls on the surface of their spores and microspores [9] , [10] , [11] , and genes encoding CYP703 homologues have been detected in these genomes [12] . Curiously, however, one of the basal vascular plants, Selaginella , contains a functional GA perception system that is mediated by a GA receptor, GIBBERELLIN-INSENSITIVE DWARF1 (GID1), and suppressor proteins (DELLAs), whereas one of the basal land plants, Physcomitrella patens , does not contain this system [13] , [14] , [15] , [16] . These observations led us to speculate that the ancestral land plants developed sporopollenin-containing outer walls on their spores, which protected the spores from dryness and ultraviolet radiation on land, in association with CYP703-like enzymes, and that GA signalling pathway then evolved to control the development of the spore outer wall via the modulation of CYP703-like expressions during the evolution from mosses to lycopods. Mutant and transgenic studies in flowering plants indicate that GAMYB preferentially modulates other aspects of reproductive developments (for example, inflorescence formation and floral organ development as well as microspore development) [1] , [7] , [8] , [17] , [18] . Moreover, considering that some GA-like substances (known as antheridiogens) are involved in the formation of sexual organs in fern gametophytes [19] , it is further likely that this GA signalling pathway that involves GAMYB regulates a broad range of reproductive processes, including (micro)spore development, in early vascular plants. In this study, we identified the functional GAMYB homologues in Selaginella moellendorffii and P. patens . In S . moellendorffii , GA treatment promoted the outer wall development on microspores, in association with the induction of CYP703 homologue. On the other hand, in P . patens with no functional GA signalling pathway, the knockouts (KOs) of two GAMYB homologues had similar abnormalities in spore development and showed the transcriptional reduction of CYP703 homologues, supporting that the regulation of CYP703 by GAMYB is conserved among land plant lineages. Moreover, the KOs failed to develop male organs, instead ectopically forming female organs. On the basis of these results, we propose that GA signalling might have merged to regulate this pre-existing GAMYB-based system in reproductive development. In silico screening for GAMYB-like genes To test our hypothesis, we first searched for homologues of GAMYB in mosses and lycopods. A survey of public genomic phytozome database showed that the model moss P. patens has two GAMYB-like genes, PpGAMYB1 and PpGAMYB2 , whereas the model lycopod S. moellendorffii contains a single GAMYB-like gene, SmGAMYB ( Fig. 1a ; Supplementary Fig. S1a ). A comparative analysis of these GAMYB-like genes with GAMYBs in flowering plants revealed that these homologues shared three conserved regions (BOX1, BOX2 and BOX3) in addition to a R2R3 DNA-binding domain and a putative microRNA 159 target site ( Fig. 1a ; Supplementary Fig. S1b ), which are ubiquitous in GAMYBs of flowering plants [18] , [20] . 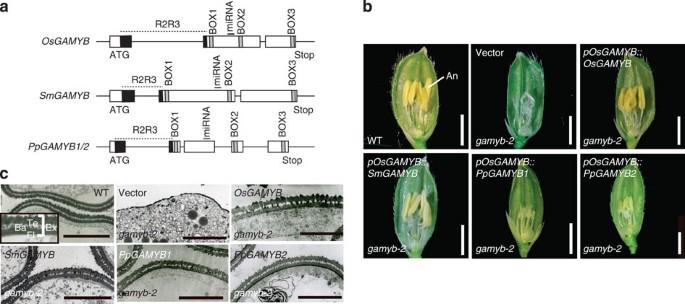Figure 1: Conserved molecular function ofSmGAMYBandPpGAMYBs. (a) The exon/intron structure ofOsGAMYBandGAMYBhomologues. The coding regions and introns are symbolized by boxes and lines, respectively. Black box, R2R3 DNA-binding domain; grey boxes, BOX1–3 domains; black line above gene structure, putative miR159 target site. (b,c), Flower (b) and the microspore outer wall (exine) (c) of wild-type (WT) rice plants and of transgenic plants transformed with empty vector,OsGAMYBandGAMYBhomologues in the ricegamyb-2background (n>11). Inset indicates the magnification of WT exine layer. Scale bars indicate 2 mm inband 5 μm inc. An, anther; Ba, bacula; Ex, exine; Fl, foot layer; Te, tectum. Figure 1: Conserved molecular function of SmGAMYB and PpGAMYB s. ( a ) The exon/intron structure of OsGAMYB and GAMYB homologues. The coding regions and introns are symbolized by boxes and lines, respectively. Black box, R2R3 DNA-binding domain; grey boxes, BOX1–3 domains; black line above gene structure, putative miR159 target site. ( b , c ), Flower ( b ) and the microspore outer wall (exine) ( c ) of wild-type (WT) rice plants and of transgenic plants transformed with empty vector, OsGAMYB and GAMYB homologues in the rice gamyb-2 background ( n >11). Inset indicates the magnification of WT exine layer. Scale bars indicate 2 mm in b and 5 μm in c . An, anther; Ba, bacula; Ex, exine; Fl, foot layer; Te, tectum. Full size image A previous study of the CYP703 family reported that three homologues of this protein were present in P. patens (PpCYP703B1–3) and one was present in S. moellendorffii [12] (SmCYP703C1). Molecular characterization of SmGAMYB and PpGAMYBs To test the function of these putative GAMYB homologues, we fused the GAMYB coding sequence (CDS) from each species to the rice GAMYB ( OsGAMYB ) promoter, and transformed these constructs into a rice loss-of-function mutant, gamyb-2 . As previously reported, the observations by the transmission electron microscopy (TEM) revealed that the wild type (WT) plants developed microspores with a normal exine consisting of three layers in the anthers (tectum, bacula and foot layer [1] ; Fig. 1b and inset of Fig. 1c ), whereas gamyb-2 plants transformed with an empty vector developed microspores with a defective exine consisting of a single layer, resulting in shrunken and whitened anthers that lacked pollen grains relative to yellow anthers of WT ( Fig. 1b,c ). The gamyb-2 plants transformed with OsGAMYB developed microspores with a normal exine structure that consisted of three layers ( Fig. 1c ). Anther development was partially rescued in transgenic plants carrying SmGAMYB ( Fig. 1b ). The anthers of these plants were slightly whitened ( Fig. 1b ), and the microspores exhibited a normal exine consisting of three layers ( Fig. 1c ). In PpGAMYB1 and PpGAMYB2 transgenic lines, anther development was also partially rescued ( Fig. 1b ), which exhibited microspores with a normal exine ( Fig. 1c ). We also examined whether the CYP703 homologues in P . patens and S . moellendorffii had sporopollenin biosynthetic activity. For this analysis, we used SmCYP703C1 (the sole homologue detected in S . moellendorffii ) and PpCYP703B2 (the dominant gene of three PpCYP703B homologues; see below). A defect in exine structure in pollen of the rice loss-of-function cyp703a3 mutant was fully rescued by introduction of the CDS for SmCYP703C1 under the control of the rice CYP703A3 promoter, and at least partially rescued by introduction of PpCYP703B2 with the same rice promoter ( Supplementary Fig. S2 ). Taken together, our results show that the biological function of GAMYB and CYP703 homologues for the outer wall development is conserved among the land plant lineage. However, the level of activity varied among each family member, at least in rice cells. To further confirm the function of the GAMYB homologues in the GA signalling pathway in rice cells, we compared the expression pattern in the anthers of OsGAMYB transgenic plants with those of SmGAMYB or PpGAMYB2 transgenic plants, using two-color microarrays hybridized with RNA isolated from rice gamyb-2 anthers as a common reference ( Supplementary Methods , Data are available at Gene Expression Omnibus, accession code: GSE32652.). Most OsGAMYB-regulated genes that were expressed in response to OsGAMYB expression ( x axis) were also, at least partially, regulated at the transcriptional level by the SmGAMYB and PpGAMYB2 expression ( y axis; Supplementary Fig. S3a,b and Supplementary Data 1 ). The transcriptional recovery by SmGAMYB expression was more tightly correlated to OsGAMYB-mediated modulation than was the transcriptional recovery by PpGAMYB2 expression (correlation coefficient; 0.84 in Supplementary Fig. 3a and 0.71 in Supplementary Fig. 3b ). The difference in correlation coefficient agrees with the rescued phenotype of transgenic rice plants ( Fig. 1b,c ). Consistently, the expression of an OsGAMYB target gene, CYP703A3 , which was hardly detected in the gamyb-2 background, was complemented by the introduction of SmGAMYB to a similar or higher degree than it was by OsGAMYB , whereas PpGAMYB s partially restored CYP703A3 expression, with PpGAMYB2 having a stronger effect than did PpGAMYB1 ( Supplementary Fig. S3c ). Together, these results indicate that SmGAMYB can almost completely substitute, and PpGAMYB proteins can partially substitute, for OsGAMYB in the GA signalling pathway of rice anther development. Role of GA in microspore development of S. moellendorffii During the divergence of basal vascular plants including lycopods from the moss lineage, a GA receptor, GID1 and DELLA repressors were established as key components for GA perception system in association with a functional GA biosynthetic pathway, indicating the occurrence of the entire GA signalling pathway [13] , [14] . However, the biological function of GA in basal vascular plants has been unclear, as GA treatment does not cause any developmental defects at the vegetative stage, such as increased stem or leaf elongation, in Selaginella [13] . Therefore, we hypothesized that, in such basal vascular plants, GA may be exclusively involved in the outer wall development of microspores via GAMYB. Quantitative RT–PCR analysis using various tissues of S. moellendorffii revealed SmGAMYB and SmCYP703C1 were preferentially expressed in the reproductive organs, strobili ( Fig. 2a,b ). The microsporangium in the strobili of a heterosporous lycophyte, S . moellendorffii, is an orthologous organ of the anther of flowering plants. Microspores within the microsporangium correspond to pollen grains of flowering plants. Previous observations suggested that GA signalling mediated by GAMYB is important for anther and pollen development in flowering plants [1] , [7] , [8] . Therefore, we next performed an in situ hybridization experiment to examine the spatiotemporal expression of SmGAMYB and SmCYP703C1 during microsporangium development ( Fig. 2c–e ). During the transition from premeiosis to young microspore stage, the expression of these genes was mainly limited to the tapetal cells and microspores in a pattern similar to that of a GA biosynthesis gene, GA3 oxidase ( SmGA3ox ; Fig. 2c–e ), where the sporopollenin material is produced for the outer wall development [9] , [10] , [11] , [21] , [22] , [23] . Considering that GAMYBs , CYP703A s and GA biosynthesis genes in flowering plants are also co-expressed in the tapetal cells and microspores [1] , [8] , [12] , [24] , [25] , [26] , these observations indicate that SmGAMYB activity in these tissues of Selaginella is required to mediate GA signalling during the outer wall formation of microspores. 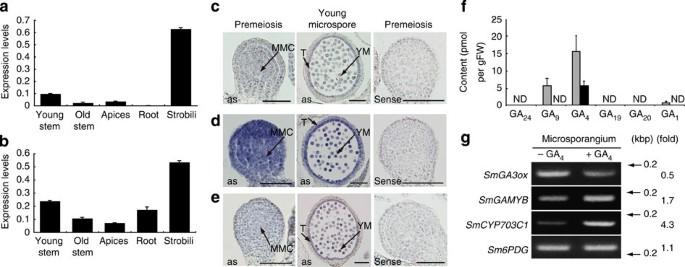Figure 2: The spatioexpression pattern ofSmGAMYBandSmCYP703C1in microspore development ofS. moellendorffii. (a,b) Quantitative RT–PCR analysis ofSmGAMYB(a) andSmCYP703C1(b) in different tissues. Data are shown as the mean values±s.d. (n=3). (c–e)In situhybridization ofSmGA3ox(c),SmGAMYB(d) andSmCYP703C1(e) on microsporangium at the premeiosis stage (left and right) and young microspore stage (middle). Scale bars, 50 μm. as, anti-sense; MMC, microspore mother cell; T, tapetal cell; YM, young microspore. (f) Endogenous GA content ofS. moellendorffiimicrosporangia (grey) and young stems (black). Data are shown as the mean values±s.d. (n=3). FW, fresh weight; ND, no expected product was detected. (g)SmGA3ox,SmGAMYBandSmCYP703C1expression in response to GA4treatment in microsporangium. Number on the right side of each panel indicates the expression ratio in GA4treatment versus in Mock control, estimated by Image J software. Figure 2: The spatioexpression pattern of SmGAMYB and SmCYP703C1 in microspore development of S. moellendorffii . ( a , b ) Quantitative RT–PCR analysis of SmGAMYB ( a ) and SmCYP703C1 ( b ) in different tissues. Data are shown as the mean values±s.d. ( n =3). ( c – e ) In situ hybridization of SmGA3ox ( c ), SmGAMYB ( d ) and SmCYP703C1 ( e ) on microsporangium at the premeiosis stage (left and right) and young microspore stage (middle). Scale bars, 50 μm. as, anti-sense; MMC, microspore mother cell; T, tapetal cell; YM, young microspore. ( f ) Endogenous GA content of S. moellendorffii microsporangia (grey) and young stems (black). Data are shown as the mean values±s.d. ( n =3). FW, fresh weight; ND, no expected product was detected. ( g ) SmGA3ox , SmGAMYB and SmCYP703C1 expression in response to GA 4 treatment in microsporangium. Number on the right side of each panel indicates the expression ratio in GA 4 treatment versus in Mock control, estimated by Image J software. Full size image To further verify the importance of GA in spore wall formation, we analysed the endogenous GA level in the microsporangium. We detected a 13 non-hydroxylated bioactive GA, GA 4 , in microsporangia, and, to a lesser extent, in young stems ( Fig. 2f ). Because bioactive GA negatively regulates the expression of some GA biosynthetic genes, including GA3ox , and positively regulates the expression of GAMYB and CYP703A in flowering plants [1] , [8] , [13] , we decided to examine the expression levels of these homologues in the presence and absence of GA 4 . Application of GA 4 to the microsporangium suppressed the expression of SmGA3ox , whereas it induced SmGAMYB and SmCYP703C1 ( Fig. 2g ). As is the case in the pollen grains of flowering plants, these results demonstrate that the GA response is present in the microspores of S . moellendorffii . Then, we examined the effect of GA 4 or a GA biosynthesis inhibitor, uniconazole, which inhibits a step of the GA biosynthesis pathway that is catalysed by ent -kaurene oxidase [27] , on the exospore development of S . moellendorffii microspores using scanning electron microscopy (SEM). The SEM observations revealed that the outer exospore of microspores in mock-treated plants was formed as numerous sporopolleninous projections ( Fig. 3a ), the material of which originates exclusively from the tapetum and microspores [11] , [23] . The heights of the outer exospore projections of GA 4 -treated microspores were significantly greater than those of mock-treated microspores, whereas the microspores treated with uniconazole produced less and shorter outer exospore projections than did the mock-treated microspores ( Fig. 3a,b ). Such defects in outer exospore projections were not detected in the microspores of plants that were simultaneously treated with GA 4 and uniconazole, and the number and height of the outer exospore projections of the microspores of these plants were similar to those of GA 4 -treated plants ( Fig. 3a,b ). Moreover, a similar phenotype was induced upon treatment with another GA biosynthesis inhibitor, prohexadione-calcium, which inhibits another step of the GA biosynthesis pathway catalysed by GA3ox [28] , and was rescued by co-treatment with GA 4 ( Fig. 3a,b ), strongly suggesting that these phenomena depend on a GA deficiency. These results show that, similar to flowering plants, basal vascular plants require the GA signalling pathway to promote the development of the microspore outer exospore wall. 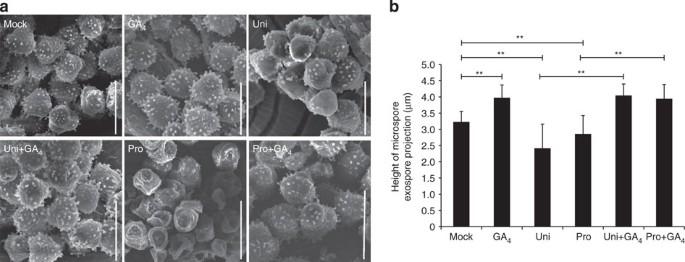Figure 3: Effects of GA4or GA biosynthesis inhibitors on the exospore projection of the microspore surface ofS. moellendorffii. (a) SEM images of the exospore of microspores developed by the treatment of GA4or GA biosynthesis inhibitors inS. moellendorffii. Scale bars, 50 μm. Pro, prohexadione-calcium; Uni, uniconazole. (b) The height of the exospore projection on the microspore following treatment with GA4or GA biosynthesis inhibitors. Measurements were made on SEM micrographs using Image J software, and data represent mean values±s.d. (Mock control:n=230; GA4:n=219; uniconazole (Uni):n=321; prohexadione-calcium (Pro):n=89; GA4and uniconazole (Uni+GA4):n=178; GA4and prohexadione-calcium (Pro+GA4):n=91). **P<0.01; Tukey's test. Figure 3: Effects of GA 4 or GA biosynthesis inhibitors on the exospore projection of the microspore surface of S. moellendorffii . ( a ) SEM images of the exospore of microspores developed by the treatment of GA 4 or GA biosynthesis inhibitors in S. moellendorffii . Scale bars, 50 μm. Pro, prohexadione-calcium; Uni, uniconazole. ( b ) The height of the exospore projection on the microspore following treatment with GA 4 or GA biosynthesis inhibitors. Measurements were made on SEM micrographs using Image J software, and data represent mean values±s.d. (Mock control: n =230; GA 4 : n =219; uniconazole (Uni): n =321; prohexadione-calcium (Pro): n =89; GA 4 and uniconazole (Uni+GA 4 ): n =178; GA 4 and prohexadione-calcium (Pro+GA 4 ): n =91). ** P <0.01; Tukey's test. Full size image Role of PpGAMYBs in spore development of P . patens We first examined the expression pattern of PpGAMYBs to estimate the biological function of PpGAMYB s in P . patens , which has no functional GA perception system and GA biosynthetic pathway [13] , [14] ( Fig. 4a,b ). P . patens develops protonemata colony from spores, and then differentiates gametophores with haploid leafy shoots and root-like rhizoids from a fraction of the protonema [29] ( Fig. 4c and Supplementary Fig. S4a,b ). Subsequently, at the shoot apex of the gametophore, the archegonium and antheridium ( Fig. 4d,e ), which contain an egg and sperm cells, respectively, develop, and an egg cell is fertilized by a sperm cell [29] . Finally, the resulting zygote develops a sporophyte that contains a spore-producing tissue, the sporangium [29] ( Fig. 4f ). Quantitative RT–PCR analysis revealed that transcripts for PpGAMYB s, PpCYP703B1 and PpCYP703B2 were present in various tissues of gametophore, but not in the protonema, whereas PpCYP703B3 transcript was not present in any tested tissues ( Fig. 4a,b ). In sporangium of the sporophyte, PpGAMYB2 and PpCYP703B2 were expressed more strongly than the other transcripts analysed ( Fig. 4a,b ), indicating that they might have a dominant role in sporangium development. The spatiotemporal expression pattern of PpGAMYB1 and PpGAMYB2 was further examined by introducing the β-glucuronidase ( GUS ) reporter gene just upstream of the stop codon of each gene ( Fig. 4c–f ). During the young gametophore stage, GUS activity in the PpGAMYB1-GUS and PpGAMYB2-GUS plants was mainly detected in the shoot apices and partially in the rhizoid ( Fig. 4c ). During the reproductive stage, the GUS signal was detected in the developing archegonium and antheridium ( Fig. 4d,e ). After the start of sporogenesis, the GUS signal in these two lines was detected in the sporangium ( Fig. 4f ). In situ hybridization revealed that PpGAMYB1 and PpCYP703B1 were co-expressed more strongly in spores than in spore sac cells ( Supplementary Fig. S5a,b ; insets). In contrast, the transcripts of PpGAMYB2 and PpCYP703B2 , the predominantly expressed genes, co-localized in spore sac cells of the sporangium ( Supplementary Fig. S5c,d ; insets), which correspond to tapetal cells in flowering plants [29] . 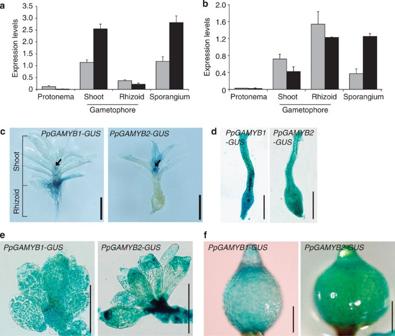Figure 4: Expression pattern ofPpGAMYBsandPpCYP703Bsin various tissues ofP. patens. (a) Quantitative RT–PCR analysis ofPpGAMYB1(grey) andPpGAMYB2(black) in different tissues ofP. patens. Data represent mean values±s.d. (n=3). (b) Quantitative RT–PCR analysis ofPpCYP703B1(grey) andPpCYP703B2(black) in different tissues ofP. patens. Data represent mean values±s.d. (n=3). (c–f) GUS expression pattern in the leafy gametophore (c), archegonium (d), antheridia (e) and sporangium (f) of PpGAMYB1-GUS (left) and PpGAMYB2-GUS (right) reporter lines. Arrows mark the shoot apex. Scale bars indicate 1 mm inc, 100 μm ind,e, and 200 μm inf. Figure 4: Expression pattern of PpGAMYBs and PpCYP703Bs in various tissues of P. patens . ( a ) Quantitative RT–PCR analysis of PpGAMYB1 (grey) and PpGAMYB2 (black) in different tissues of P. patens . Data represent mean values±s.d. ( n =3). ( b ) Quantitative RT–PCR analysis of PpCYP703B1 (grey) and PpCYP703B2 (black) in different tissues of P. patens . Data represent mean values±s.d. ( n =3). ( c – f ) GUS expression pattern in the leafy gametophore ( c ), archegonium ( d ), antheridia ( e ) and sporangium ( f ) of PpGAMYB1-GUS (left) and PpGAMYB2-GUS (right) reporter lines. Arrows mark the shoot apex. Scale bars indicate 1 mm in c , 100 μm in d , e , and 200 μm in f . Full size image To further investigate the function of PpGAMYB s, we generated KO lines of PpGAMYB1 and PpGAMYB2 ( PpGAMYB1 -KO and PpGAMYB2 -KO) using homologous recombination. There were no morphological and growth defects in the protonemata and gametophores in each single KO line ( Supplementary Fig. S4a–c ). On the other hand, after 4 or 5 weeks of antheridium and archegonium induction, antheridium formation was strongly disturbed in PpGAMYB2 -KO, whereas archegonium formation was promoted in PpGAMYB -KOs ( Fig. 5a ). Most PpGAMYB2 -KO plants displayed ectopic archegonium formation at the site of antheridium formation, and a similar, but milder, trend was seen in PpGAMYB1 -KO ( Fig. 5b ). Moreover, some abnormal antheridia that were light brown were observed in these KOs (asterisks in Fig. 5c ). Consistent with these abnormal antheridium phenotypes, the number of sporophytes was reduced ( Fig. 5d,e ), while developed sporophytes appeared to be normal in PpGAMYB -KOs ( Fig. 5f ). 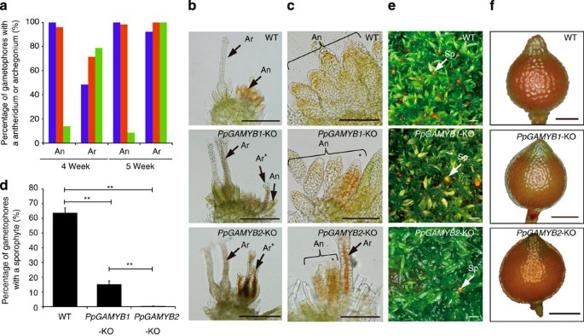Figure 5: Effect ofPpGAMYBknockout on reproductive development inP. patens. (a) Quantification of antheridium and archegonium formation in the WT (blue),PpGAMYB1-KO (red) andPpGAMYB2-KO (green) knockout lines. The percentage of gametophores containing antheridia or archegonia relative to the total number of gametophores after 4 or 5 weeks in antheridium/archegonium induction conditions is given (n>37). An, antheridium; Ar, archegonium. (b,c) Morphology of antheridia and archegonia in WT (upper),PpGAMYB1-KO (middle) andPpGAMYB2-KO (lower)P. patens. Ar*, ectopic archegonium. Scale bars indicate 250 μm inband 100 μm inc. Asterisks mark the abnormal antheridium. (d) Quantification of sporangium formation in the WT andPpGAMYBknockout lines. The percentage of gametophores containing a sporangium relative to the total number of gametophores after 3 months under antheridium/acrhegonium induction conditions is given (n=4). **P<0.01; Tukey's test. (e,f) Morphology of mature gametophores (e) and a sporophyte (f) of the WT (upper),PpGAMYB1-KO (middle) andPpGAMYB2-KO (lower). Sp, sporophyte. Scale bars indicate 1 mm ineand 0.3 mm inf. Figure 5: Effect of PpGAMYB knockout on reproductive development in P . patens . ( a ) Quantification of antheridium and archegonium formation in the WT (blue), PpGAMYB1 -KO (red) and PpGAMYB2 -KO (green) knockout lines. The percentage of gametophores containing antheridia or archegonia relative to the total number of gametophores after 4 or 5 weeks in antheridium/archegonium induction conditions is given ( n >37). An, antheridium; Ar, archegonium. ( b , c ) Morphology of antheridia and archegonia in WT (upper), PpGAMYB1 -KO (middle) and PpGAMYB2 -KO (lower) P. patens . Ar*, ectopic archegonium. Scale bars indicate 250 μm in b and 100 μm in c . Asterisks mark the abnormal antheridium. ( d ) Quantification of sporangium formation in the WT and PpGAMYB knockout lines. The percentage of gametophores containing a sporangium relative to the total number of gametophores after 3 months under antheridium/acrhegonium induction conditions is given ( n =4). ** P <0.01; Tukey's test. ( e , f ) Morphology of mature gametophores ( e ) and a sporophyte ( f ) of the WT (upper), PpGAMYB1 -KO (middle) and PpGAMYB2 -KO (lower). Sp, sporophyte. Scale bars indicate 1 mm in e and 0.3 mm in f . Full size image Within the sporophyte, however, there were differences in the surfaces of the spores in each KO ( Fig. 6a,b ), and the number of spores in each KO was less than in the WT ( Table 1 ). The SEM observations of mature spores revealed that WT spores produced well-developed spiny projections on their surface, whereas development of such projections occurred incompletely in PpGAMYB -KOs, resulting in a smoother surface ( Fig. 6a,b ) and a higher frequency of collapsed spores (arrowheads in Fig. 6a ). We noticed that the PpGAMYB2- KO had a more severe phenotype than the PpGAMYB1- KO, which is consistent with PpGAMYB2 being expressed at a higher level than PpGAMYB1 in WT sporangium ( Fig. 4a ). The collapsed spores observed in PpGAMYB -KOs suggest that the structural and physical protection against the vacuum condition of SEM analysis might be reduced in PpGAMYB -KOs spores, compared with WT spores. We next treated spores with a solution of acetic anhydride and sulphuric acid, which generally disrupts all spore/pollen content except for the exospore/exine by hydrolysis and esterification (acetolysis) [30] , [31] . The spores in PpGAMYB -KOs, especially in the PpGAMYB2 -KO, were easily damaged by acetolysis treatment (percentage of acetolysis-sensitive spores in PpGAMYB1 -KO, 23.32±2.68%; PpGAMYB2 -KO, 60.33±8.97%; and WT, 14.63±3.21%; Fig. 6c and Table 1 ). Considering that the effect of acetolysis is dominantly reflected by the exospore content, the result suggests that dynamic alternation of exospore structure occurs in these KOs. We also observed the ultrastructure of spore walls developed in PpGAMYB -KOs by the TEM and revealed structural differences in PpGAMYB -KOs. As described previously [32] , [33] , the spore wall in the WT consists of four layers, the intine, inner exospore, outer exospore and perine ( Fig. 6d,e ). Among these layers, the perine layer, which contributes to the formation of projections of spores, was severely defective in the KO spores, especially in PpGAMYB2 -KO ( Fig. 6d,e ). Moreover, the continuous outer exospore structure was sporadically interrupted in PpGAMYB1 -KO (arrowheads in Fig. 6d ), and often in PpGAMYB2 -KO, whereas there were no obvious defects in the inner exospore and intine layers of PpGAMYB -KOs ( Fig. 6d,e ). These observations are in good agreement with previous reports that the sporopollenin material for perine and exospore is mainly supplied from the spores and spore sac cells [11] , [34] , where PpGAMYB s and PpCYP703B s were expressed ( Supplementary Fig. S5 ). 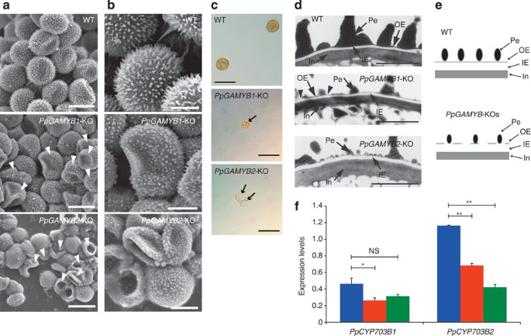Figure 6: Effect ofPpGAMYBknockout lines on spore development inP. patens. (a,b) SEM images (a) and their magnification (b) of spores developed in WT (upper),PpGAMYB1-KO (middle) andPpGAMYB2-KO (lower) ofP. patens(n=15). Arrowheads indicate collapsed spores. Scale bars indicate 25 μm inaand 10 μm inb. (c) Spore morphology after the acetolysis incubation. Arrows indicate the debris of spores. Scale bars, 50 μm. (d) The outer wall structure of WT,PpGAMYB1-KO andPpGAMYB2-KO spores. Arrowheads indicate the interrupted domains of the outer exospore. Scale bars, 2 μm. IE, inner exospore; In, intine; OE, outer exospore; Pe, perine. (e) Diagrams of spore wall structure in the WT (upper) andPpGAMYB-KOs (lower). The abnormal wall structures inPpGAMYB-KOs are marked by dotted lines. (f)PpCYP703Bsexpression in WT (blue),PpGAMYB1-KO (red) andPpGAMYB2-KO (green) sporangia. Data represent mean values±s.d. (n=3). **P<0.01; *P<0.05; N-S, not significant; Student'st-test (two-tailed). Figure 6: Effect of PpGAMYB knockout lines on spore development in P . patens . ( a , b ) SEM images ( a ) and their magnification ( b ) of spores developed in WT (upper), PpGAMYB1 -KO (middle) and PpGAMYB2 -KO (lower) of P. patens ( n =15). Arrowheads indicate collapsed spores. Scale bars indicate 25 μm in a and 10 μm in b . ( c ) Spore morphology after the acetolysis incubation. Arrows indicate the debris of spores. Scale bars, 50 μm. ( d ) The outer wall structure of WT, PpGAMYB1 -KO and PpGAMYB2 -KO spores. Arrowheads indicate the interrupted domains of the outer exospore. Scale bars, 2 μm. IE, inner exospore; In, intine; OE, outer exospore; Pe, perine. ( e ) Diagrams of spore wall structure in the WT (upper) and PpGAMYB -KOs (lower). The abnormal wall structures in PpGAMYB -KOs are marked by dotted lines. ( f ) PpCYP703Bs expression in WT (blue), PpGAMYB1 -KO (red) and PpGAMYB2 -KO (green) sporangia. Data represent mean values±s.d. ( n =3). ** P <0.01; * P <0.05; N-S, not significant; Student's t -test (two-tailed). Full size image Table 1 Characterization of the spores of PpGAMYB knockouts. Full size table Consistent with the abnormal perine and exospore layers of PpGAMYB -KOs, the expression of PpCYP703B1 and PpCYP703B2 was lower in the sporangia of the KOs than in those of the WT ( Fig. 6f ). The suppression level of PpCYP703B1 was significantly greater in PpGAMYB1 -KO than in PpGAMYB2 -KO, whereas that of PpCYP703B2 was greater in PpGAMYB2 -KO than in PpGAMYB1 -KO ( Fig. 6f ). The expression level of PpCYP703B2 in PpGAMYB2 -KO was decreased to one-third of that in the WT, whereas that in PpGAMYB1 -KO was almost half of that in the WT ( Fig. 6f ). The suppression level of PpCYP703B1 was not significantly less than that of PpCYP703B2 in PpGAMYB1 -KO and PpGAMYB2 -KO ( Fig. 6f ). However, the level of PpCYP703B1 decreased to a greater degree in PpGAMYB1 -KO than in PpGAMYB2 -KO, and the opposite was the case for PpCYP703B2 ( Fig. 6f ). This corresponds with the co-expression pattern of PpGAMYB1 and PpCYP703B1 , and PpGAMYB2 and PpCYP703B2 in sporangium ( Supplementary Fig. S5 ). In the 1-kb promoter region of PpCYP703B2, a paralogue that is predominantly expressed in sporangia ( Fig. 4b ), there are four putative GAMYB-binding sequences with a TAAC core sequence [35] (filled circles in Supplementary Fig. S6a ). Among these DNA fragments, the P4 fragment effectively inhibited the interaction between the truncated PpGAMYB2 containing the DNA-binding domain and the authentic GAMYB-binding sequence of rice α-amylase1A , RAmy1A ( Supplementary Fig. S6b ). The P4 fragment contains two putative GAMYB-binding sequences ( Supplementary Fig. S6a ), and a DNA fragment mutagenized at the lower GAMYB core sequence (mP4-2) failed to inhibit its interaction ( Supplementary Fig. S6b,c ), suggesting that PpCYP703B2 is a direct target of PpGAMYB. Taken together, these data indicate that the direct regulation of CYP703 by GAMYB has an important role in the development of the spore/pollen outer walls in moss and flowering plants. In this study, we demonstrated that, in S . moellendorffii and P . patens, as in flowering plants, GAMYB homologues regulate CYP703 expression to promote the development of the outer walls of spores/microspores, even although the GA signalling and biosynthesis pathways do not exist in P . patens . Further, since these GAMYB homologues in non-flowering plants at least partially compensated for the lack of OsGAMYB in the rice GA signalling pathway, we propose the following evolutional model of the GA signalling pathway ( Fig. 7 ): The common ancestor of basal land plants before the separation of the mosses had GAMYB-mediated regulation in the proto-tapetal cells (spore sac cells) and spores for spore outer wall formation. At this stage, the GAMYB-mediated regulation of spore outer wall formation was independent of the GA signalling pathway, as the GA signalling pathway had not yet been established [13] , [14] . Consistent with this hypothesis, it is reported that the disruption of multiple DELLA -like genes in P . patens did not affect the plant's life cycle [14] , and that the disruption of PpCPS/KS , which encodes ent -kaurene synthase, an enzyme essential for GA synthesis in flowering plants, did not result in abnormal spore development [36] . In the next step, the common ancestor of basal vascular plants before the separation of the lycopsids acquired GA biosynthesis and GA signalling pathways to regulate the pre-existing GAMYB-mediated system, leading to the establishment of the GA signalling pathway via GAMYB. This conclusion is further supported by the fact that GA is important for microspore exospore wall development and SmCYP703C1 expression in Selaginella ( Figs 2g and 3 ). 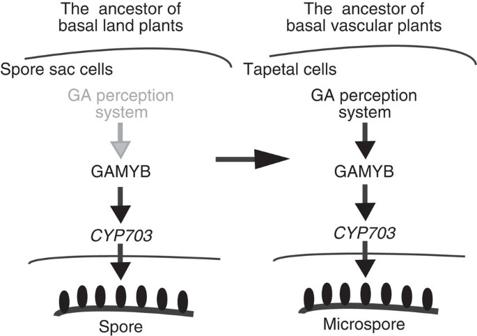Figure 7: Evolutional model of GA-mediated outer wall formation. Before the establishment of GA perception system (left), the common ancestor of basal land plants had GAMYB-mediated regulation for spore outer wall formation. In the next evolutional step (right), the common ancestor of basal vascular plants acquired GA biosynthesis and GA signalling pathways to regulate the pre-existing GAMYB-mediated system, leading to the establishment of the GA signalling pathway via GAMYB. Grey letter indicates a loss of indicated molecular system. Figure 7: Evolutional model of GA-mediated outer wall formation. Before the establishment of GA perception system (left), the common ancestor of basal land plants had GAMYB-mediated regulation for spore outer wall formation. In the next evolutional step (right), the common ancestor of basal vascular plants acquired GA biosynthesis and GA signalling pathways to regulate the pre-existing GAMYB-mediated system, leading to the establishment of the GA signalling pathway via GAMYB. Grey letter indicates a loss of indicated molecular system. Full size image PpGAMYB2- KO failed to induce antheridia, and instead exhibited ectopic archegonium formation ( Fig. 5a,b ). This result suggests that GAMYB is involved in the formation of the gametophytic sexual organs in P . patens . GA and its derivatives are known to modulate the formation/development of sexual organs during the reproductive stage in some tree ferns and flowering plants [19] . Although the downstream factors in this sexual organ developmental process in fern plants have not been identified [37] , these observations suggest that, after the establishment of the GA perception system, the first function of the GA perception system may have been to promote sexual organ formation and spore/pollen development at the reproductive stage via GAMYB. In other words, the GA signalling pathway may have originally arisen to regulate reproduction. There is a working model that could explain the occurrence of GA control of the GAMYB system in the course of plant evolution. Similar to the ancestors of land plants, P. patens , which develops a parasitic sporophyte on the gametophyte, has a gametophyte-dominant life cycle, whereas vascular plants, including S. moellendorffii, have a sporophyte-dominant life cycle [29] . The evolutional transition from a gametophyte- to a sporophyte-dominant life cycle and the subsequent adaptation to the land environment have increased the complexity of the sexual reproduction system: for example, the transition from spore sac cells to tapetal cells, and the transition from homospory to heterospory. Thus, to complete the sexual reproduction in a novel manner, the GA perception system and the pre-existing GAMYB might be used by the early vascular plants, including S. moellendorffii . Particularly, in male reproductive development, this GA-dependent control of GAMYB might allow the coordinated development of various cell types so that it can be synchronized with female reproductive development. Plant materials and chemical treatment The rice cultivars Oryza sativa cv Nipponbare (WT); gamyb-2 (mutant of GAMYB protein) and cyp703a3-1 (mutant of CYP703A3 protein) were used in this study [1] , [7] . The strain of P. patens , WT62, and the same strain of S. moellendorffii as one of previous report [13] were used as the WT. The plants except P. patens were grown at 28 °C in a greenhouse. P. patens on the sterile peat pellets was cultured at 28 °C under the continuous light for 3 weeks, and then moved to 15 °C under 8 h light and 16 h dark conditions to induce antheridium/acrhegonium. For the expression analysis using microsporangia of the S. moellendorffii , the detached strobili were placed in a solution of 150 mM sucrose containing 10 −5 M GA 4 or ethanol for 12 h at 22 °C, and then microsporangia were collected from the strobili. For the ultrastructure studies using microspores of S . moellendorffii treated with mock (1/1,000th EtOH), 10 −4 M GA 4 , 10 −6 M uniconazole, 10 −4 M prohexadione-calcium, 10 −4 M GA 4 and 10 −6 M uniconazole, or 10 −4 M GA 4 and 10 −4 M prohexadione-calcium, samples were sprayed three times weekly with the respective solution, after the development of the first strobili. At the end of 1 month, a sample of strobili was collected for the SEM observation. Plasmid construction and plant transformation The sequences of the primers used in this study are listed in Supplementary Table S1 . The PCR fragments were sequenced to confirm that no mutations were introduced. For the complementation of GAMYB and CYP703 homologues in P . patens and S . moellendorffii , the CDS of each gene was amplified from complementary DNA of P . patens gametophores or S . moellendorffii strobili using the indicated primer sets. The resulting PCR fragments of GAMYB homologues contained a Bam HI site at its 5′ end and a Xho I site at its 3′ end, whereas those of CYP703 homologues contained a Nco I site at its 5′ end and a Sma I or EcoR V site at its 3′ end. These resulting PCR fragments were then cloned into the pCR4 Blunt-TOPO vector (Invitrogen). After that, each construct was excised at its enzyme sites, and the resulting fragment was ligated into pOsGAMYB ∷ nos-pCAMBIA1380 or pOsCYP703A3 ∷ nos-pCAMBIA1380 plasmid carrying the hygromycin resistance cassette. These chimeric constructs were introduced into Agrobacterium tumefaciens strain EHA105 and used to infect rice callus according to previous report [38] . To produce the PpGAMYB constructs used to generate P . patens KO lines, the 5′- and 3′-flanking sequence of each PpGAMYB -coding region was cloned from genomic DNA of P . patens using the corresponding primers. The resulting 5′- and 3′-fragment of each PpGAMYB contained Eco RV and Sma I site at its 5′ and 3′ ends, and was then introduced into Eco RV and Sma I site of the pTN186 and pTN182 vectors in the correct orientation, generating PpGAMYB1-pTN186 and PpGAMYB2-pTN182. To obtain GAMYB-GUS fusion transformants, a genomic region of each PpGAMYB from the middle to the last codon of the CDS, was introduced in-frame 5′ to the GUS gene of pTN85. The genomic fragment containing the 3′-flanking region of each PpGAMYB gene was inserted into the 3′-region of the NPTII expression cassette of this plasmid. To transform these plasmids into P . patens , polyethylene glycol-mediated transformation was performed essentially as described [30] , using 10 μg of linearized plasmid. Stable transformants were screened by Southern hybridization using a probe that detected the homologous region of the transgene. Microscopy and phenotypic analyses For GUS staining, tissues were transferred to microcentrifuge tubes containing a solution of 50 mM sodium phosphate, pH 7.0, 7% methanol, and 1 mM 5-bromo-4-chloro-3-indolyl-β- D -glucuronide for 12 h at 37 °C. Stained tissues were destained with an ethanol series. For in situ hybridization, plant materials were fixed in 4% (w/v) paraformaldehyde and 0.25% (v/v) glutaraldehyde in 0.1 M sodium phosphate buffer, pH 7.4, overnight at 4 °C, dehydrated through a graded ethanol series followed by a t -butanol series, and finally embedded in Paraplast Plus (Sherwood Medical). Microtome sections (8–10 μm thick) were mounted on glass slides treated with silane. To produce the gene-specific probes, each DNA fragment was generated by PCR using complementary DNA and the specific primers. The resulting DNA fragments were introduced between Xho I and EcoR I site of the pBluescript II SK+ and pBluescript II KS+ vectors, and were then transcribed in vitro under T7 promoter with T7 RNA polymerase (Invitrogen) using the DIG RNA labeling kit (Roche). Hybridization and immunological detection of the hybridized probes were performed essentially as described [39] . The primer sequences used in this study are listed in Supplementary Table S1 . For observations by TEM, plant samples were vacuum infiltrated three times for 10 min with fixative (4% paraformaldehyde and 1% glutaraldehyde in 0.05 M cacodylate buffer, pH 7.4). Procedures for ultrastructural studies were essentially the same as described [40] . For observations by SEM, fresh microspores/spores were placed on specimen stubs using adhesive carbon tape. The samples were gold coated with Pt and Pd in an ion sputter (E-1030, Hitachi), and imaged using SEM (S-3000N microscope, Hitachi). For the acetolysis experiments, spores were collected in a tube and incubated in 9:1 (v/v) mixture of acetic anhydride and sulphuric acid at 70 °C for 20 min. After the incubation, spores were transferred on a glass slide and observed by the light microscopy (Olympus). Endogenous GA analysis Extraction and determination of GA of S. moellendorffii microsporangia and young stems were performed using a liquid chromatography–tandem mass chromatography system (AQUITY UPLC System/Quattro Premier XE, Waters) as described [41] . Data were processed by MassLynx software with QuanLynx (version 4.0, Waters). RNA isolation and RT–PCR analysis Total RNA was isolated from tissue samples using RNeasy plant minikit (Qiagen). The first strand of cDNA was synthesized from 1 μg of total RNA using an Omniscript reverse transcription kit (Qiagen). Transcripts were quantified by RT–PCR or real-time RT–PCR analyses using one-twentieth of the resulting cDNA as template. Real-time RT–PCR was performed with the LightCycler system (Roche) with the SYBR Green PCR kit (Qiagen). For RT–PCR analysis, an adequate volume of each cDNA sample was used for PCR amplification with different numbers of cycles (20–35 cycles) to confirm the linear range of PCR amplification for each gene. The results were confirmed using three independent biological replicates. The Sm6PGD , PpUbiquitin or OsActin1 genes were used as internal standards for normalizing cDNA concentration variations. The primer sequences used in this study are listed in Supplementary Table S1 . Accession Codes: The microarray data have been deposited in the Gene Expression Omnibus under accession code GSE32652 . How to cite this article: Aya, K. et al . The Gibberellin perception system evolved to regulate a pre-existing GAMYB-mediated system during land plant evolution. Nat. Commun. 2:544 doi: 10.1038/ncomms1552 (2011).